Degradation of MONOCULM 1 by APC/CTAD1regulates rice tillering A rice tiller is a specialized grain-bearing branch that contributes greatly to grain yield. The MONOCULM 1 ( MOC1 ) gene is the first identified key regulator controlling rice tiller number; however, the underlying mechanism remains to be elucidated. Here we report a novel rice gene, Tillering and Dwarf 1 ( TAD1 ), which encodes a co-activator of the anaphase-promoting complex (APC/C), a multi-subunit E3 ligase. Although the elucidation of co-activators and individual subunits of plant APC/C involved in regulating plant development have emerged recently, the understanding of whether and how this large cell-cycle machinery controls plant development is still very limited. Our study demonstrates that TAD1 interacts with MOC1, forms a complex with OsAPC10 and functions as a co-activator of APC/C to target MOC1 for degradation in a cell-cycle-dependent manner. Our findings uncovered a new mechanism underlying shoot branching and shed light on the understanding of how the cell-cycle machinery regulates plant architecture. Rice is one of the most important cereal crops in the world and provides the staple food for more than half of the world's population. Rice grain yields are determined by many factors, among which tiller number is generally regarded as the determining factor because tillers are specialized branches bearing panicles. Rice tillering has been intensively investigated over the past decade owing to its agronomic importance and significant progress has been made in identifying genes that regulate rice tillering [1] . Among them, the MOC1 gene is the first identified key regulator that controls rice tiller number [2] . MOC1 encodes a member of the plant-specific GRAS family, an ortholog of LS in tomato and LAS in Arabidopsis [2] , [3] , [4] . MOC1 controls the initiation and outgrowth of axillary meristems at both vegetative and reproductive stages. As a result, the loss-of-function of MOC1 affects both tiller and panicle branches. The other two important regulators, LAX1 and LAX2, are also involved in the formation of axillary meristems throughout the development of rice plants [5] , [6] . Considering the additive effects of lax1 moc1 , lax2 moc1 and lax1 lax2 double mutants, MOC1 , LAX1 and LAX2 may function in different regulatory pathways [5] , [6] , which implies a complicated mechanism underlying the axlliary meristem formation in rice. The cell cycle is one of the most important biological processes owing to its crucial role in regulating the growth and development of an organism. Timely coordinated degradation of specific regulators ensures unidirectional and irreversible progression of the cell cycle [7] . Two ubiquitin ligases, the anaphase-promoting complex/cyclosome (APC/C) and the Skp1/Cullin/F-box (SCF), act complementarily to accomplish basic cell-cycle control [7] . The genetic, biochemical and structural studies have demonstrated that the APC/C is a 1.5-megadalton E3 ligase assembled from 13 different subunits [8] . The targeting specificity and activation of the APC/C are defined by either of the two adaptor proteins, Cdc20 or Cdh1, and the docking protein, APC10/Doc1 [7] . As a co-activator, Cdh1 controls cell-cycle progression and genome stability by binding the APC/C complex, recognizing and recruiting specific substrates, which include mitotic cyclins, mitotic kinases, proteins involved in chromosome segregation, DNA replication proteins and transcription factors [9] . In plants, the orthologs of Cdh1 , CELL CYCLE SWITCH52 genes ( CCS52A and CCS52B ), were first isolated from Medicago truncatula nodule and root libraries, respectively [10] , [11] . Further studies demonstrated that CCS52A functions conservatively in dicot species. In Medicago, CCS52A has been reported to control endoreduplication in leaf petioles and nodules [10] , [11] . In Arabidopsis , besides the role of CCS52A in endoreduplication for the control of leaf size and the trichome branching, it is also required for meristem maintenance in roots [12] , [13] , [14] . In tomato, CCS52A-regulated endoreduplication affects fruit growth [15] . Similar to Cdh1 that directly targets cyclins and is inhibited by early mitotic inhibitor 1 (Emi1) in animals [7] , CCS52A has also been demonstrated to be inhibited by ULTRAVIOLET-B-INSENSITIVE4 (UVI4) and GIGAS CELL1 (GIG1)/OMISSION OF SECOND DIVISION1 (OSD1) and to target CYCA2;3 for regulating endoreduplication in Arabidopsis [16] , [17] , [18] . In addition, individual APC/C subunits, APC2, APC4, APC6, APC8, APC13 and CDC27, have been found to have critical roles in gametogenesis or embryogenesis in Arabidopsis [19] , [20] , [21] , [22] , [23] . APC10 has been shown to regulate leaf and vascular development in Arabidopsis [24] , [25] . In rice, OsAPC6 may be involved in the control of plant height [26] . Although the elucidation of co-activators and individual subunits of the plant APC/C complex involved in regulating plant development have emerged recently, the mechanism of whether and how this large cell-cycle machinery targets different substrates and controls plant growth and development is still unclear. Here, we report the isolation and functional characterization of a novel rice tillering mutant, tillering and dwarf 1 ( tad1 ), which shows increased tillers and reduced plant height. TAD1 encodes a Cdh1-type activator of APC/C, an ortholog to CCS52A in dicots [10] , [11] . During the cell-cycle progression, TAD1 shows an oscillating expression pattern with a higher level in the G1-phase. We found that TAD1 interacts with MOC1, forms a complex with OsAPC10 and functions as a co-activator of APC/C to target MOC1 for degradation in a cell-cycle-phase-dependent manner. Cloning and characterization of the TAD1 gene To gain more insight into the molecular basis of rice tillering, we identified and characterized a rice tillering mutant, tad1 . The tad1 mutant showed an increased tiller number, a reduced plant height, and twisted leaves and panicles ( Fig. 1a–e ). Using 2,200 F 2 plants generated from the cross between MH63 and tad1 , the candidate gene was narrowed down to a 22.5-kb region between the markers RM523 and S1273 on chromosome 3 ( Fig. 1f and Supplementary Table S1 ). Within this region, there exist four predicted genes ( Supplementary Table S2 ). Sequence analysis revealed a single base substitute (TGG→TGA) at the second exon of LOC_Os03g03150 in tad1 , which produces a premature stop codon ( Fig. 1f and Supplementary Fig. S1 ). To verify whether LOC_Os03g03150 is the corresponding TAD1 gene, we carried out a genetic complementation test by transferring the plasmid containing the entire TAD1 coding region, 2,721-bp 5′-upstream and 1,827-bp 3′-downstream sequences ( Supplementary Fig. S2a ), into the tad1 plant. All ten transgenic lines showed complementation of the tad1 phenotype ( Supplementary Fig. S2b ) indicating that LOC_Os03g03150 is the TAD1 gene and the premature mutation is responsible for the phenotypes of the tad1 mutant plant. 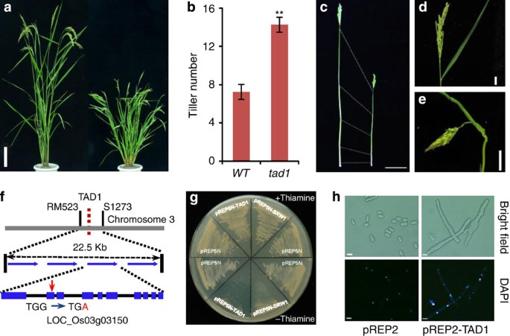Figure 1: Map-based cloning and characterization ofTAD1. (a) The phenotypes of the wild type (left) andtad1(right). Scale bar, 10 cm. (b) Comparison of tiller number between the wild type (left) andtad1(right). Values are means with s.e. (n=35 plants). The double asterisks represent the significant difference determined by thet-test atP<0.01. (c) Comparison of plant height between the wild type (left) andtad1(right). Scale bar, 10 cm. (d) The panicle and flag leaf of the wild type. Scale bar, 3 cm. (e) The panicle and flag leaf oftad1. Scale bar, 3 cm. (f) Map-based cloning ofTAD1.TAD1was mapped in a 22.5-kb DNA region between the molecular markers, RM523 and S1273, on chromosome 3. Blue arrows represent the four predicted open reading frames, the red arrow indicates a single base substitution in the second exon of LOC_Os03g03150 intad1and the red letter represents the mutation of G to A that results in a stop codon TGA. (g) Growth ofS. pombetransformed with pREP5N-TAD1, pREP5N-SRW1 and the empty vector pREP5N in the presence and absence of thiamine. (h) Phenotypes ofS. pombecells transformed with pREP2-TAD1 and the empty vector pREP2 in the absence of thiamine. Scale bars, 10 μm. Figure 1: Map-based cloning and characterization of TAD1 . ( a ) The phenotypes of the wild type (left) and tad1 (right). Scale bar, 10 cm. ( b ) Comparison of tiller number between the wild type (left) and tad1 (right). Values are means with s.e. ( n =35 plants). The double asterisks represent the significant difference determined by the t -test at P <0.01. ( c ) Comparison of plant height between the wild type (left) and tad1 (right). Scale bar, 10 cm. ( d ) The panicle and flag leaf of the wild type. Scale bar, 3 cm. ( e ) The panicle and flag leaf of tad1 . Scale bar, 3 cm. ( f ) Map-based cloning of TAD1 . TAD1 was mapped in a 22.5-kb DNA region between the molecular markers, RM523 and S1273, on chromosome 3. Blue arrows represent the four predicted open reading frames, the red arrow indicates a single base substitution in the second exon of LOC_Os03g03150 in tad1 and the red letter represents the mutation of G to A that results in a stop codon TGA. ( g ) Growth of S. pombe transformed with pREP5N-TAD1, pREP5N-SRW1 and the empty vector pREP5N in the presence and absence of thiamine. ( h ) Phenotypes of S. pombe cells transformed with pREP2-TAD1 and the empty vector pREP2 in the absence of thiamine. Scale bars, 10 μm. Full size image Sequence analysis revealed that TAD1 encodes a putative cell-cycle switch protein, belonging to a Cdh1 group of APC/C co-activators, which include fission yeast SRW1/STE9 [27] , [28] , budding yeast CDH1/HCT1 [29] , [30] , Drosophila FZR1 [31] , Medicago MtCCS52A [10] , Arabidopsis AtCCS52A [12] , [13] , and mouse and human Cdh1 [32] , [33] , [34] ( Supplementary Fig. S1 ). Phylogenetic analysis showed that TAD1 is highly homologous to MtCCS52A in Medicago and AtCCS52A1 in Arabidopsis [35] , which have been reported to have crucial roles in endoreduplication [10] , [13] , [14] . The TAD1 -deduced amino-acid sequence contains several conserved domains, including seven WD repeats, C-box, CSM, RVL and IR motifs ( Supplementary Fig. S1 ). Previous work showed that the plant protein MtCCS52A is an ortholog of Cdh1. Induced overexpression of MtCCS52A elicited a severe phenotype manifested by growth inhibition and extreme elongation of the yeast cells [10] . To demonstrate the functional similarity of TAD1 to these proteins, the TAD1 complementary DNA (cDNA) was cloned into the pREP5N or pREP2 yeast vector and expressed in the absence of thiamine. As shown in Fig. 1g,h , overexpression of TAD1 in Schizosaccharomyces pombe also resulted in growth arrest and cell enlargement. Moreover, flow cytometry analyses of the suspension cell lines of wild type and tad1 revealed a significant increase in the number of the cells in the G2/M-phase of the cell cycle in the tad1 mutant line ( Fig. 2a ). These results demonstrated that TAD1 is involved in regulating the exit of mitosis and we therefore conclude that TAD1 is indeed a functional cell-cycle switch protein homologous to Cdh1 . 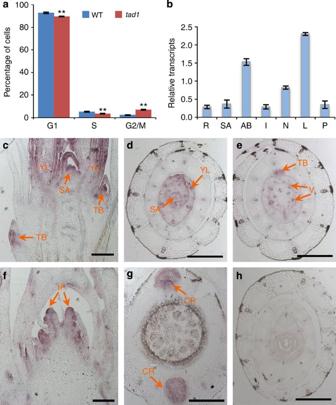Figure 2: Expression patterns ofTAD1. (a) Flow cytometric analysis of the cell-cycle profiles of the wild type (WT) and mutant (tad1). Nuclei released from the wild-type andtad1suspension cells were stained with 4,6-diamidino-2-phenylindole (DAPI) for flow cytometry analysis. The percentage of cells in each phase of the cell cycle was quantified by the ModFit LT software. Values are means with s.e. (n=4). The double asterisks indicate the significant difference determined by the two-tailedt-test atP<0.01. (b)TAD1transcript levels in various organs, including roots (R), shoot apexes of seedlings (SA), axillary buds (AB), internodes (I), nodes (N), young leaves (L) and young panicles (P). Values are means with s.d. of three independent experiments. (c–h)TAD1expression patterns revealed by messenger RNAin situhybridization. YL, young leaf; TB, tiller bud; IF, inflorescence; SA, shoot apex; CR, crown root; V, vascular bundle. Arrows in (c–g) indicate theTAD1expression sites. (h) Thein situhybridization result withTAD1sense probe. Scale bars, 500 μm. Figure 2: Expression patterns of TAD1 . ( a ) Flow cytometric analysis of the cell-cycle profiles of the wild type (WT) and mutant ( tad1 ). Nuclei released from the wild-type and tad1 suspension cells were stained with 4,6-diamidino-2-phenylindole (DAPI) for flow cytometry analysis. The percentage of cells in each phase of the cell cycle was quantified by the ModFit LT software. Values are means with s.e. ( n =4). The double asterisks indicate the significant difference determined by the two-tailed t -test at P <0.01. ( b ) TAD1 transcript levels in various organs, including roots (R), shoot apexes of seedlings (SA), axillary buds (AB), internodes (I), nodes (N), young leaves (L) and young panicles (P). Values are means with s.d. of three independent experiments. ( c–h ) TAD1 expression patterns revealed by messenger RNA in situ hybridization. YL, young leaf; TB, tiller bud; IF, inflorescence; SA, shoot apex; CR, crown root; V, vascular bundle. Arrows in ( c – g ) indicate the TAD1 expression sites. ( h ) The in situ hybridization result with TAD1 sense probe. Scale bars, 500 μm. Full size image Expression patterns of TAD1 Real-time PCR analysis showed that TAD1 is expressed ubiquitously in the examined rice organs, including roots, shoot apices, axillary buds, internodes, nodes, and young leaves and panicles, but more abundant in young leaves, axillary buds and nodes ( Fig. 2b ). The tissue-specific expression pattern of TAD1 was further examined by messenger RNA in situ hybridization. TAD1 was predominantly expressed in the leaf primordia and young leaves ( Fig. 2c,d ), tiller buds ( Fig. 2c,e ), inflorescence promordia ( Fig. 2f ), and crown root promordia ( Fig. 2g ). In addition, TAD1 expression was detected in vascular bundles at the unenlongated stem ( Fig. 2e ). To further examine whether the expression of TAD1 is dependent on cell-cycle progression, we synchronized the rice suspension cells with aphidicolin, a reversible inhibitor of the G1/S-phase. The efficiency of synchronization was determined by flow cytometry analysis ( Fig. 3a ). After being treated with aphidicolin for 18 h, the suspension cells were released from aphidicolin, and then at an interval of 3 h the treated cells were analysed flow cytometrically and TAD1 transcript levels were measured. The results revealed that TAD1 has an oscillated expression pattern during the cell-cycle progression, showing a higher level in the G1-phase and a lower level in the S- and G2/M-phases ( Fig. 3b ). The efficiency of the synchronization culture was further confirmed by the G2- to M-phase markers OsCDKB;2 and CYCB1;1 [36] , [37] ( Supplementary Fig. S3 ). 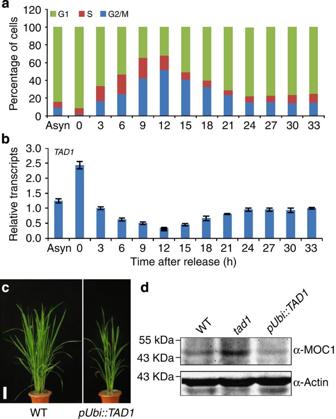Figure 3: Expression of TAD1 during the cell-cycle progression and phenotypes ofTAD1-overexpressing transgenic plants. (a) Flow cytometry analysis of asynchronously growing (Asyn) and synchronized rice suspension cells after release from aphidicolin at indicated time points. The number of cells in the G1-, S- or G2/M-phase is given as percentages of the total cell population.(b)TAD1expression levels during the cell-cycle progression. (c) Phenotypes ofTAD1-overexpressing transgenic plants. Scale bar, 10 cm. (d) Immunodetection of endogenous MOC1 levels in the wild-type,tad1andTAD1-overexpressing transgenic plants. Figure 3: Expression of TAD1 during the cell-cycle progression and phenotypes of TAD1 -overexpressing transgenic plants. ( a ) Flow cytometry analysis of asynchronously growing (Asyn) and synchronized rice suspension cells after release from aphidicolin at indicated time points. The number of cells in the G1-, S- or G2/M-phase is given as percentages of the total cell population. (b) TAD1 expression levels during the cell-cycle progression. ( c ) Phenotypes of TAD1 -overexpressing transgenic plants. Scale bar, 10 cm. ( d ) Immunodetection of endogenous MOC1 levels in the wild-type, tad1 and TAD1 -overexpressing transgenic plants. Full size image TAD1 may regulate tillering upstream of MOC1 MOC1 has been previously demonstrated to function as a key regulator of tiller formation and development in rice [2] . The overexpression of MOC1 resulted in similar phenotypes to that of the tad1 mutant plant, such as more tillers and reduced plant height [2] , whereas TAD1 -overexpressing transgenic plants showed a reduced tiller number ( Fig. 3c and Supplementary Fig. S4a,b ), a similar phenotype to moc1 [2] . These reciprocal similarities suggested that TAD1 and MOC1 may coordinately regulate rice tillering. We therefore examined the MOC1 protein levels in wild-type, tad1 and TAD1 -overexpressing plants. As shown in Fig. 3d and Supplementary Fig. S4c , MOC1 accumulated to a higher level in tad1 , but is reduced in TAD1 -overexpressing plants in comparison with the wild-type plants, implying that TAD1 most likely controls rice tillering through regulating MOC1. TAD1 interacts directly with MOC1 The APC complex has been known to target its substrates conferred by co-activators (Cdc20 and Cdh1) through recognition of destruction motifs, predominantly the destruction box (D-box) and KEN-box [38] , [39] . The amino-terminal D-box has been shown to have a critical role in directing the APC complex when recognizing its substrates [38] . Sequence analysis revealed that MOC1 harbours a typical D-box at the N-terminal ( Fig. 4a ). Therefore, it is very likely that MOC1 and TAD1 directly interact to control rice tillering. To investigate the interaction between MOC1 and TAD1, we carried out coimmunoprecipitation experiments by coexpressing TAD1–FLAG and MOC1–green fluorescent protein (MOC1–GFP) fusion proteins in protoplasts generated from rice suspension cells. The result showed that the MOC1–GFP fusion protein could capture the TAD1–FLAG fusion protein, suggesting an in vivo interaction between MOC1 and TAD1 ( Fig. 4b ). The interaction was further examined through a bimolecular fluorescence complementation (BiFC) analysis. As shown in Fig. 4c , when the full-length cDNAs of TAD1 and MOC1 were introduced into rice protoplasts simultaneously, the fluorescence signal was detected in the nucleus, indicating that TAD1 can directly interact with MOC1 in the nucleus. Furthermore, when two conserved residues, arginine and leucine, of the D-box at the N-terminal were changed into alanine ( Fig. 4a ), the MOC1 protein was unable to interact with TAD1, demonstrating that the D-box is indispensable for the interaction between MOC1 and TAD1 ( Fig. 4c ). In addition, a series of truncated TAD1 proteins were generated to determine the domains that are essential for the interaction with MOC1 via the BiFC analysis ( Fig. 4d ). The results showed that the N-terminal 203 amino acids of TAD1 are sufficient to interact with MOC1. However, the truncation mutant at C456, which lacks the N-terminal 67 amino acids of TAD1, could not recognize MOC1 in the BiFC analysis, suggesting that the 67-amino-acid N-terminal of TAD1 appears to be essential for its interaction with MOC1 ( Fig. 4e ). 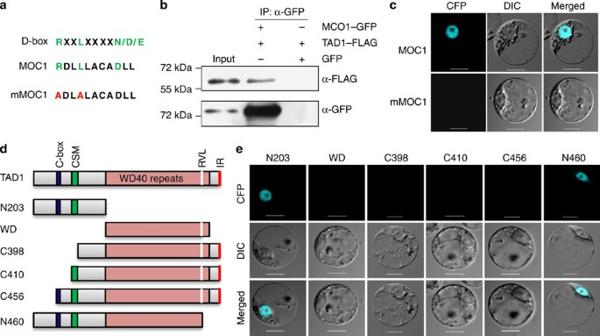Figure 4: Determination of the interaction between TAD1 and MOC1 by coimmunoprecipitation and BiFC assays. (a) The conserved D-box motif at the MOC1 N-terminal and its mutated construct (mMOC1). (b)In vivointeraction between TAD1 and MOC1 revealed by the coimmunoprecipitation assay. (c) BiFC analysis of interaction between MOC1 and TAD1 in rice protoplasts. Scale bars, 10 μm. (d) Schematic representation of the truncated TAD1 proteins. Blue box refers to C-box, green to CSM, pink to WD repeats, white to RVL, and red to IR. (e) BiFC analyses ofin vivointeraction between MOC1 and truncated TAD1 proteins indicated in (d). Scale bars, 10 μm. Figure 4: Determination of the interaction between TAD1 and MOC1 by coimmunoprecipitation and BiFC assays. ( a ) The conserved D-box motif at the MOC1 N-terminal and its mutated construct (mMOC1). ( b ) In vivo interaction between TAD1 and MOC1 revealed by the coimmunoprecipitation assay. ( c ) BiFC analysis of interaction between MOC1 and TAD1 in rice protoplasts. Scale bars, 10 μm. ( d ) Schematic representation of the truncated TAD1 proteins. Blue box refers to C-box, green to CSM, pink to WD repeats, white to RVL, and red to IR. ( e ) BiFC analyses of in vivo interaction between MOC1 and truncated TAD1 proteins indicated in ( d ). Scale bars, 10 μm. Full size image MOC1 is the target of TAD1 for degradation Cdh1 has been shown to act as a co-activator of APC/C and to function through recruiting substrates to APC/C for degradation [7] . The fact that TAD1 interacts with MOC1 and MOC1 is accumulated in the tad1 mutant plant suggests that MOC1 may be the target of TAD1 for degradation in rice. We therefore performed several experiments to test this possibility. We examined the degradation of endogenous MOC1 in rice plant extracts using a cell-free degradation system, which is an effective in vitro degradation assay system supporting the proteasome-mediated pathway [40] , [41] . To analyse protein degradation, the cell-free degradation buffer consisting of components required for proteasome-mediated degradation was used to extract total proteins from plants. The degradation dynamics of plant proteins in the extracts were monitored by immunoblotting. As shown in Fig. 5a , when MOC1 protein levels in rice suspension cells were detected upon treatment with AEBSF (serine proteases inhibitor), Pepstatin A (acid protease inhibitor) or MG132 (proteasome inhibitor), respectively, the degradation of MOC1 was exclusively inhibited by the treatment with MG132, indicating that MOC1 was degraded in a proteasome-dependent manner. Next, we performed an in vitro ubiquitination assay using MOC1-GFP transgenic calli. The result showed that the endogenous MOC1 protein could be polyubiquitinated ( Fig. 5b ). Finally, we examined the degradation of expressed recombinant MOC1 monitored by the cell-free degradation assay. GST-MOC1 proteins were expressed and purified from Escherichia coli , and then added to the wild-type and tad1 extracts. The results indicated that the degradation rate of MOC1 is slower in the tad1 mutant than in the wild-type plant extracts ( Fig. 5c ). Consistently, when the MOC1 proteins containing a mutated D-box motif were incubated with wild-type extracts, the degradation of MOC1 was attenuated, showing that MOC1 is degraded in a D-box-dependent manner ( Fig. 5c ). Moreover, when MOC1 was overexpressed in the wild-type or tad1 mutant cultured cells, respectively, the dynamic degradation of MOC1 was altered in tad1 . In the wild-type background, the MOC1 was degraded after 30 min and to a very low level after 60 min, but in the tad1 background it underwent only a slight degradation ( Fig. 5d ). Collectively, these results demonstrated that MOC1 is directly targeted by TAD1 as a substrate for degradation in vivo and its D-box at the N-terminus functions as an APC/C TAD1 recognition motif for degradation. 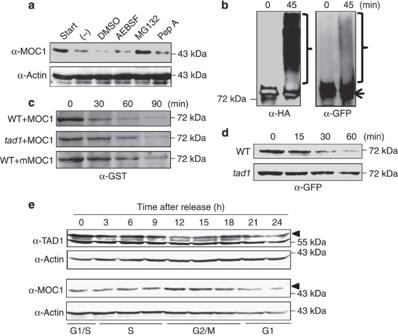Figure 5: TAD1 targets MOC1 in a cell-cycle phase-dependent manner. (a) Cell-free degradation assay showing the proteasome-dependent degradation of MOC1. Detection of Actin served as an internal control. (b)In vitroubiquitination assay of immunopurified MOC1-GFP in the presence of recombinant HA–ubiquitin. The arrow represents unmodified MOC1-GFP, and the brace refers to ubiquitination-modified MOC1-GFP. (c)In vitrocell-free degradation assay showing the delayed degradation of expressed recombinant GST-MOC1 intad1and GST-mMOC1 in the wild type. The protein levels at different time points were detected by western blotting using the GST antibodies. (d) Dynamic degradation of MOC1-GFP in the wild-type (WT) andtad1transgenic calli. Immunoblotting by the GFP antibodies showed the remaining protein levels of MOC1-GFP at different time points. (e) Profiles of TAD1 and MOC1 protein levels during the cell-cycle progression. The cell-cycle phase is determined by flow cytometry at different time points after release from synchronized rice suspension cells as indicated in the scheme at bottom. Black triangles refer to the TAD1 or MOC1 protein in the immunoblots, respectively. Figure 5: TAD1 targets MOC1 in a cell-cycle phase-dependent manner. ( a ) Cell-free degradation assay showing the proteasome-dependent degradation of MOC1. Detection of Actin served as an internal control. ( b ) In vitro ubiquitination assay of immunopurified MOC1-GFP in the presence of recombinant HA–ubiquitin. The arrow represents unmodified MOC1-GFP, and the brace refers to ubiquitination-modified MOC1-GFP. ( c ) In vitro cell-free degradation assay showing the delayed degradation of expressed recombinant GST-MOC1 in tad1 and GST-mMOC1 in the wild type. The protein levels at different time points were detected by western blotting using the GST antibodies. ( d ) Dynamic degradation of MOC1-GFP in the wild-type (WT) and tad1 transgenic calli. Immunoblotting by the GFP antibodies showed the remaining protein levels of MOC1-GFP at different time points. ( e ) Profiles of TAD1 and MOC1 protein levels during the cell-cycle progression. The cell-cycle phase is determined by flow cytometry at different time points after release from synchronized rice suspension cells as indicated in the scheme at bottom. Black triangles refer to the TAD1 or MOC1 protein in the immunoblots, respectively. Full size image We further investigated whether the degradation of MOC1 by TAD1 occurs during cell-cycle progression by examining their relative levels in synchronized rice suspension cells. As shown in Fig. 5e , MOC1 was accumulated to a higher level at the G2/M-phase, while TAD1 was at a lower level at the same phase, implying that TAD1 degrades MOC1 at the G1-phase. TAD1 forms a protein complex with OsAPC10 for targeting MOC1 Recent studies have revealed that Cdh1 and Doc1 (APC10) can act as the D-box coreceptors in budding yeast [42] , [43] . We therefore isolated OsAPC10 cDNAs from rice seedlings to investigate whether OsAPC10 can coordinate with TAD1 to recognize MOC1 in rice. OsAPC10 and TAD1 cDNAs were cloned into BiFC vectors, which were subsequently used to cotransfect rice protoplasts for analysing their interaction. 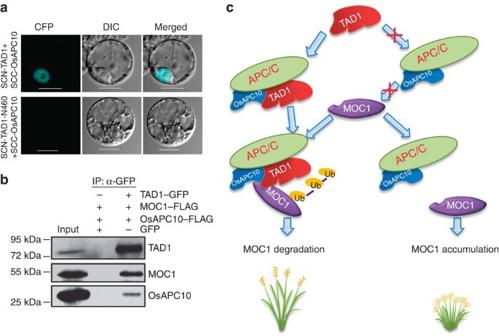Figure 6: The APC/CTAD1complex-mediated degradation of MOC1. (a) BiFC assays indicated the interaction between TAD1 and OsAPC10 in the nucleus of rice protoplasts. The N-terminal 460 amino acids of TAD1 served as a negative control for the BiFC assay. Scale bars, 10 μm. (b) MOC1 coimmunoprecipitated with TAD1 and OsAPC10in vivo.IP, immunoprecipitation. (c) A working model of rice tillering regulated by the APC/CTAD1complex. Figure 6a shows that OsAPC10 interacts with TAD1 in vivo and their interaction occurs in the nucleus of rice protoplasts. Furthermore, we coexpressed TAD1, MOC1 and OsAPC10 proteins in the rice protoplasts and performed coimmunoprecipitation experiments to detect their interaction. We found that MOC1 can indeed form a protein complex with TAD1 and OsAPC10 in vivo ( Fig. 6b ). Therefore, it is very likely that TAD1 recruits MOC1 to APC/C, and OsAPC10 is also involved in recognizing and targeting MOC1 for further degradation. Figure 6: The APC/C TAD1 complex-mediated degradation of MOC1. ( a ) BiFC assays indicated the interaction between TAD1 and OsAPC10 in the nucleus of rice protoplasts. The N-terminal 460 amino acids of TAD1 served as a negative control for the BiFC assay. Scale bars, 10 μm. ( b ) MOC1 coimmunoprecipitated with TAD1 and OsAPC10 in vivo. IP, immunoprecipitation. ( c ) A working model of rice tillering regulated by the APC/C TAD1 complex. Full size image Among the rice plant architecture determinants such as plant height, tiller number, tiller angle and panicle morphology, rice tiller has received particular attention because of its grain-bearing feature that contributes directly to grain yields [44] . Although several key regulators, such as MOC1, LAX1 and LAX2, were successively identified in the past decade, our understanding on rice tillering is still fragmented. In this study, we identified a component of the cell-cycle machinery, TAD1, which forms the APC/C TAD1 complex and functions as a key regulator of tillering. Our study demonstrates that TAD1 can specifically recruit MOC1 by interacting with OsAPC10 and then degrade MOC1 to maintain an appropriate protein level of MOC1 to control rice tillering. In the absence of TAD1 function, MOC1 fails to be recruited to the APC/C for degradation, resulting in an accumulation of endogenous MOC1 proteins and thus an increase in tiller number in the tad1 mutant plant ( Fig. 6c ). In animals, in addition to its essential role involved in cell-cycle progression, the APC/C has also been reported recently to target different substrates in non-mitotic cells such as neurons, muscle cells and lens fibre cells [45] . In the ventral nerve cord of Caenorhabditis elegans , the APC/C complex regulates synaptic strength by affecting the number of glutamate receptors on the postsynaptic side [46] . In Drosophila , APC/C Cdh1 regulates presynaptic organization and synaptic size by targeting liprin-α for degradation [47] . In mammals, knockdown of Cdh1 leads to increased axon and disrupted axonal patterning [48] . Further studies showed that Cdh1 targets two key development regulators, inhibitor of DNA binding 2 (Id2) and the transcription corepressor ski-related novel protein N (SnoN), for degradation in regulating the axonal pattern [49] , [50] . In plants, however, whether APC/C targets the key regulators of plant development other than conserved cell-cycle regulators is still unknown. MOC1 is the first identified target of Cdh1-type co-activator of APC/C other than cyclins in plants. Loss-of-function of TAD1 disrupts normal plant architecture in rice, which is comparable to the axon phenotypes in mammals. In animals, Cdh1 functions vary during the cell-cycle progression, targeting different substrates in each specific cell-cycle phase [7] . Our results suggested that TAD1 may recruit MOC1 to APC/C for degradation mainly at the G1-phase. In agreement with this finding, a previous study showed that the majority of dormant bud cells were arrested in the G1-phase and these cells began to enter the S-phase after 6 to 9-h decapitation for re-activation [51] . This result indicated that cell division executes the activation of bud cells. The activity of cell division blocked in the G1-phase possibly accompanies low levels of MOC1 proteins in the dormant tiller buds. Based on the cell-cycle profile of bud cells and the function of APC/C TAD1 –MOC1, we propose that the APC/C TAD1 –MOC1 complex may act locally in tiller buds. During the cell-cycle progression of tiller bud cells, TAD1 is activated in the G1-phase, where it targets MOC1 for degradation to maintain a low level of MOC1. When tiller cells transit into the next phase, the TAD1 level is reduced, which causes MOC1 to accumulate and regain its function in controlling tillering. It is of great interest to understand how MOC1 acts in the bud cells and whether it directly regulates cell division. Our previous work showed that MOC1 encodes a transcription factor belonging to the plant-specific GRAS family, but no direct target of MOC1 has been identified in rice until now. A recent study revealed that the Arabidopsis SHR, a GRAS transcription factor, directly regulates a D-type cyclin CYCD6;1 in a cell-type- and developmental-stage-specific context [52] . Unlike animals, cyclins are particularly numerous in plants, implying their unique and more complicated roles in plant development [53] . Whether MOC1, like SHR, targets rice cyclins or not will be an important issue to be addressed in the future. Taken together, this work reports the identification and in-depth functional characterization of a specific component of the cell-cycle machinery in higher plants that regulates agronomically important traits, tillering and plant height. This finding will facilitate the genetic manipulation of plant architecture and the breeding of new varieties in agriculture in the future. Map-based cloning of TAD1 For map-based cloning of TAD1 , an F 2 mapping population was generated by a cross between tad1 and MingHui63 (MH63), a polymorphic indica variety. The TAD1 locus was primarily mapped between markers S7999 and S9681 ( Supplementary Table S1 ) on chromosome 3 using 50 F 2 tad1 mutant plants. TAD1 was further placed between markers S7999 and S9681 using 500 F 2 tad1 mutant plants, and was finally pinpointed in an interval between the markers RM523 and S1273 ( Supplementary Table S1 ). Constructs for genetic transformation To construct the gTAD1 complementation plasmid, a 7.6-kb DNA fragment, which contains a 2,721-bp 5′-upstream sequence, the entire TAD1 coding region, and a 1,827-bp 3′-downstream region, was introduced into the binary vector pCAMBIA1300. The BAC clone AC890695 was digested with Sal I and BamH I, producing a 3.0-kb fragment containing a 2,721-bp upstream sequence and partial sequence of the first exon. The remaining sequence was divided into two fragments for PCR amplification. The fragment 1 was amplified from the BAC clone AC890695 with primers gTAD1F1-F and gTAD1F1-R and the fragment 2 was amplified with primers gTAD1F2-F and gTAD1F2-R ( Supplementary Table S3 ). Finally, the three fragments were ligated into the binary vector pCAMBIA1300 to generate the complementation plasmid gTAD1 . To generate the p Ubi :: TAD1 plasmid, the TAD1 CDS was amplified using primers TAD1OE-F and TAD1OE-R ( Supplementary Table S3 ) and digested with Kpn I and Spe I for ligation into the binary vector pTCK30328 [54] . To generate the p Actin::MOC1-GFP construct, MOC1 CDS was amplified with primers MOC1GFP-F and MOC1GFP-R ( Supplementary Table S3 ), and the Sma I- Xba I-digested PCR product was then ligated into the binary vector AHLG. S. pombe strains and transformation To generate the constructs for yeast transformation, we amplified the full-length coding sequence of TAD1 with two pairs of primes, 5NTAD1-F and 5NTAD1-R, and REPTAD1-F and REPTAD1-R ( Supplementary Table S4 ). The PCR products were digested with Xho I and Not I, and ligated into pREP5N and pREP2, respectively. For transformation, the yeast cells were cultured in the YPAD liquid medium to OD 600 =0.4–0.5 at 30 °C. Plasmid DNA of 100 ng was added to 40 μl of cells for 5 min at 0 °C and then for electroporation [10] . Synchronization culture and flow cytometric analysis To generate rice suspension cells, the calli induced from the wild type and tad1 were used for liquid culture, and the cells were maintained with one medium change per week [55] . To synchronize rice suspension cells, 3-day subculture cells were treated with 20 μg ml −1 aphidicolin for 9 h and then another dosage of aphidicolin was added [56] . After being cultured in aphidicolin for a total of 18 h, cells were washed three times in the culture medium without aphidicolin and resuspended in an equal volume of the culture medium. At the time points indicated in Fig. 3a , cells were harvested for subsequent flow cytometric analysis or frozen immediately in liquid nitrogen for protein or RNA isolation. For cell-cycle profile examination, the nuclei were released as previously described [57] . Briefly, suspension cells were chopped into ice-cold Galbraith's buffer (45 mM MgCl 2 , 30 mM sodium citrate, 20 mM MOPS, 0.1% (w/v) TritonX-100, pH 7.0) using a razor blade. The resulting homogenates were passed through a 20-μm mesh to remove cellular debris. After 4,6-diamidino-2-phenylindole (2 μg ml −1 ) staining, the nuclei were subjected to flow cytometric analysis (FACSAria II flow cytometer, BD Bioscience). A total of 30,000 events were recorded and data were collected from four independent flow cytometric experiments and analysed by the ModFit LT software. Determination of expression pattern of TAD1 by real-time PCR Total RNAs from examined organs were extracted using a TRIzol kit according to the user's manual (Invitrogen). One microgram of total RNAs was treated with DNase I and used for cDNA synthesis with Superscript III RT kit (Invitrogen). Real-time PCR experiments were performed using gene-specific primers QTAD1-F and QTAD1-R ( Supplementary Table S4 ) in the reaction system of SsoFast™ EvaGreen ® supermix (BioRAD) on the CFX96 Real-time system (BioRAD) following the manufacturer's instructions. The rice Actin gene was used as an internal control. In situ hybridization RNA in situ hybridization was performed as described previously [58] with minor modification. Briefly, tissues of rice were fixed with 4% (w/v) paraformaldehyde at 4 °C overnight, followed by a series of dehydration and infiltration, and embedded in paraffin (Paraplast Plus, Sigma). The tissues were sliced into 10-μm sections with a microtome (Leica RM2145). The 400-bp (1525–1924 bp) 3′-region of TAD1 cDNA was subcloned into the pSK vector and used as the template to generate sense and antisense RNA probes. Digoxigenin-labelled RNA probes were prepared using a DIG Northern Starter Kit (Cat. No. 2039672, Roche) according to the manufacturer's instruction. Slides were observed under bright field through a microscope (Leica DMR) and photographed with a Micro colour charge-coupled device (CCD) camera (Apogee Instruments). BiFC assays in rice protoplast To construct plasmids for BiFC assays, TAD1, MOC1 and OsAPC10 were amplified by primers SCNTAD1-F and SCNTAD1-R, SCCMOC1-F and SCCMOC1-R, and OsAPC10-F and OsAPC10-R ( Supplementary Table S3 ) from the cDNAs prepared from wild-type seedlings, respectively. The PCR products were then ligated into BiFC vectors, including pSCYNE (SCN) and pSCYCE(R) (SCC) [59] , for generating SCN-TAD1, SCC-MOC1 and SCC-OsAPC10. For producing the BiFC plasmids of TAD1 truncations, the coding sequence of the corresponding truncations were amplified by specific primers ( Supplementary Table S3 ) and ligated into the SCN vector. The generated plasmids were transformed into protoplasts by PEG (polyethylene glycol)-mediated transformation method [60] . After incubation in the dark for 14 h, the CFP signals were examined and photographed under a confocal microscope at an excitation wavelength 405 nm (FluoView 1000; Olympus). Cell-free protein degradation assay For cell-free protein degradation assays, seedlings were grown in a SANYO MLR Plant Growth Chamber (MLR-351) for 14 days at 28 °C during daytime and 25 °C at night with a 16:8 (day:night) photoperiod, and calli of pActin::MOC1-GFP/LS and pActin::MOC1-GFP /tad1 were subcultured on the solid medium for 6 days at 28 °C in the dark. Total proteins were extracted in the degradation buffer (25 mM Tris-HCl, pH 7.5, 10 mM NaCl, 10 mM MgCl 2 , 4 mM PMSF, 5 mM dithiothreitol and 10 mM ATP) [41] and adjusted to equal concentrations with the degradation buffer. To monitor the degradation of the expressed recombinant GST-MOC1 and GST-mMOC1 proteins, 200 ng of the purified GST-MOC1 or GST-mMOC1 protein were added to 100-μl seedlings extracts (500 μg of total proteins) for individual assays. To detect the degradation of the native MOC1-GFP protein, 100 μl of calli extracts (500 μg of total proteins) were subject to individual assays. The reaction mixtures were incubated at 28 °C for the indicated time points. Reactions were blocked by adding the SDS–PAGE sample buffer. Samples were taken at indicated intervals for the western blotting. Mouse anti-GFP monoclonal Antibody (Cat: 11814460001, Roche) and mouse anti-GST monoclonal antibody (Cat: M20007, Abmart) were used at a 1:10,000 dilution, respectively. Antibody preparation and identification The GST-fused MOC1 or TAD1 protein was expressed in BL21 cells and affinity purified by Glutathione Sepharose 4 Fast Flow (GE Healthcare), and used to raise monoclonal antibodies in mouse and polyclonal antibody in rabbit, respectively. The resulted antibodies were purified through an IgG-affinity chromatography column (GE Healthcare) before use. The antibodies were used at a 1:1,000 dilution for western blotting. Coimmunoprecipitation To construct tag-fused transient expression plasmids for coimmunoprecipitation, the pSCYNE was modified by replacing the SCFP3A N173 with 3× FLAG to form SC-3×FLAG (SF). To generate SF-TAD1, TAD1 DNA isolated from SCN-TAD1 was digested with Spe I and Kpn I and ligated into SF. To produce SE-MOC1 and SF-MOC1, the coding sequence of MOC1 was isolated with BamH I and Kpn I digestion from SCC-MOC1 and ligated into SE and SF, respectively. To construct SF-OsAPC10 ( Supplementary Table S3 ), the coding sequence of OsAPC10 was amplified with OsAPC10-F and OsAPC10-R from the cDNA derived from wild-type seedlings. After digestion with BamH I and Kpn I, the PCR products were ligated into SF. Protoplasts generated from the suspension cells were transformed with transient expression constructs described above. After incubation of the cells at 28 °C for 14 h, proteins were extracted in the extraction buffer (50 mM Tris-HCl pH 7.5, 150 mM NaCl, 10% glycerol, 0.1% Nonidet P-40 and 1× complete protease inhibitor cocktail, Roche). The lysate was centrifuged at 17,000 g for 20 min at 4 °C. The supernatant was taken for coimmunoprecipitation experiments. Following the supplier's instruction, 30 μl of the agarose-conjugated anti-GFP monoclonal antibody (Cat: D153-8, MBL) were added into 1-mg total extracted protein and incubated in 4 °C for 3 h with gently rotating. The beads were washed three times with the extraction buffer and eluted with 30 μl of SDS–PAGE sample buffer for the western blotting analysis. Mouse anti-GFP monoclonal antibody (Cat: 11814460001, Roche) was used at a 1:10,000 dilution and mouse anti-FLAG monoclonal antibody (Cat: M20008, Abmart) was used at a 1:5,000 dilution. In vitro ubiquitination assay The callus of pActin::MOC1-GFP/LS was subcultured on solid medium for 6 days at 28 °C in the dark. Total proteins were subsequently extracted in the lysis buffer (50 mM Tris-HCl pH 7.5, 150 mM NaCl, 10% glycerol, 1% Nonidet P-40, 0.1% deoxycholate and 1× complete protease inhibitor cocktail). The MOC1-GFP protein was then purified by immnunoprecipitation using the agarose-conjugated anti-GFP monoclonal antibody (Cat: D153-8). After vigorously washing with the lysis buffer five times, the MOC1-GFP binding agarose was subjected to the ubiquitination assay system (25 mM Tris-HCl, pH 7.5, 10 mM NaCl, 10 mM MgCl 2 , 0.5 mM AEBSF, 5 mM dithiothreitol and 10 mM ATP) by adding recombinant HA–ubiquitin (Cat: U-110, Boston Biochem) and 50 μM MG132. The mixture was incubated at 28 °C for 45 min. After vigorously washing with the lysis buffer five times, the beads were eluted by SDS–PAGE sample buffer. For western blotting, the HA–ubiquitin-modified MOC1-GFP was detected by the HA monoclonal antibody (Cat: M20003, Abmart, dilution 1:5,000). How to cite this article: Xu, C. et al . Degradation of MONOCULM 1 by APC/C TAD1 regulates rice tillering. Nat. Commun. 3:750 doi: 10.1038/ncomms1743 (2012).